High-fat or ethinyl-oestradiol intake during pregnancy increases mammary cancer risk in several generations of offspring Maternal exposures to environmental factors during pregnancy influence the risk of many chronic adult-onset diseases in the offspring. Here we investigate whether feeding pregnant rats a high-fat (HF)- or ethinyl-oestradiol (EE2)-supplemented diet affects carcinogen-induced mammary cancer risk in daughters, granddaughters and great-granddaughters. We show that mammary tumourigenesis is higher in daughters and granddaughters of HF rat dams and in daughters and great-granddaughters of EE2 rat dams. Outcross experiments suggest that the increase in mammary cancer risk is transmitted to HF granddaughters equally through the female or male germ lines, but it is only transmitted to EE2 granddaughters through the female germ line. The effects of maternal EE2 exposure on offspring's mammary cancer risk are associated with changes in the DNA methylation machinery and methylation patterns in mammary tissue of all three EE2 generations. We conclude that dietary and oestrogenic exposures in pregnancy increase breast cancer risk in multiple generations of offspring, possibly through epigenetic means. Family history is a significant risk factor for breast cancer [1] . However, genetic mutations in high-penetrance genes, such as BRCA1 and BRCA2 , account for only a small proportion of familial breast cancers [2] , [3] and despite intense search, no other major genetic mutations have emerged [2] . Thus, it is possible that some familial breast cancers may be transmitted not through inheritance of gene mutations, but through mechanisms such as heritable epigenetic changes caused by in utero exposures. Maternal exposures to endocrine-disrupting chemicals (EDCs) and certain dietary factors during pregnancy have lasting effects on breast cancer risk among female offspring. We and others have shown in animal models that exposure to compounds such as oestradiol (E2) [4] , diethylstilbestrol (DES) [5] , [6] , bisphenol A [7] and high-fat (HF) intake [4] , [8] during pregnancy increases daughters' (F1 generation) mammary cancer risk. Population studies also show that women who had high birth weight [9] and daughters of women who took DES during their pregnancy [10] , [11] , [12] are at increased breast cancer risk. Pregnant women are exposed daily to various EDCs [13] . Although the causes remain unknown, serum oestrogen levels exhibit wide inter-individual variability among women undergoing a normal pregnancy [14] . Thus, there is potentially a large group of women who have been exposed to an excessive oestrogenic environment in utero and are at a high risk of developing breast cancer. The adverse effects of in utero exposures on adult health are likely mediated by epigenetic dysregulation, as the epigenome is most susceptible to perturbations in early development [15] . The precise epigenetic mechanisms involved are not known, but likely involve DNA methylation, as demonstrated by some studies [15] , [16] . DNA methylation is catalysed by DNA methyltransferases (DNMT): DNMT1 maintains methylation patterns during cell division, whereas DNMT3a and 3b induce de novo methylation [17] , [18] . In utero exposures to EDCs alter the expression of DNA methyltransferases (DNMT1, 3a and 3b) in some adult target tissues [19] , [20] , [21] , but whether the changes in DNMTs also take place in the mammary gland is unknown. More recent evidence suggests that some disease traits resulting from in utero exposures may be transmitted epigenetically through multiple generations [22] , [23] , [24] . Exposure of the developing male fetus to EDCs reduces fertility and causes prostate and kidney abnormalities that can persist for four consecutive generations [22] , [23] , [24] . In utero exposures can lead to multigenerational or transgenerational effects on disease risk. Multigenerational effects are due to direct exposure of the F1 generation embryo and F2 generation germ line present during gestation. These effects are not transmitted to the F3 generation. Transgenerational effects, in turn, are observed in at least three generations and are due to germ line transmission, as the F3 generation is not directly exposed to the environmental factor [25] . Here, we examined whether maternal exposures to HF diet or ethinyl-oestradiol (EE2) during pregnancy lead to multi- or transgenerational inheritance of mammary cancer in a carcinogen-induced rat model. Our study shows that in utero exposures to a HF diet or to EE2 lead to multi- and transgenerational increase in breast cancer risk, respectively, without any further intervening exposures. The increase in mammary cancer risk in the EE2 offspring is associated with similar alterations in DNA methylation patterns in the mammary glands of all three generations studied, suggesting that the transgenerational increase in breast cancer risk may involve epigenetic inheritance. Pregnancy exposures and breast cancer in multiple generations To test our hypothesis that maternal exposures during pregnancy to factors such as HF diet or a synthetic E2 lead to breast cancer in several generations, we fed pregnant Sprague–Dawley rats (F0) with either an AIN93G control diet or an isocaloric AIN93G-based HF diet, containing 43% energy from corn oil, throughout gestation. Another group of pregnant rats was fed AIN93G diet supplemented with 0.1 p.p.m. EE2 from day 14 to day 20 of pregnancy. F1 females were mated with F1 males from the same group to produce the F2 generation. The F3 generation was produced in the same manner ( Supplementary Fig. S1a ). No sibling mating was carried out. The F1, F2 and F3 offspring were maintained on the AIN93G control diet for the duration of the experiment. HF or EE2 diet of the F0 dams did not affect litter size or pups' weights in any of the three generations studied ( Supplementary Figs S2 and S3 ). Mammary tumours were induced in F1–F3 female offspring by carcinogen exposure on postnatal day (PND) 50. Daughters (F1 generation) of dams exposed to HF or EE2 during pregnancy had higher mammary tumour incidence and multiplicity ( Figs 1a,b and 2a,b ) compared with controls (HF: P =0.049, t -test and P =0.010, t -test; EE2: P =0.029, log-rank test and P =0.011, t -test), as reported before [4] . 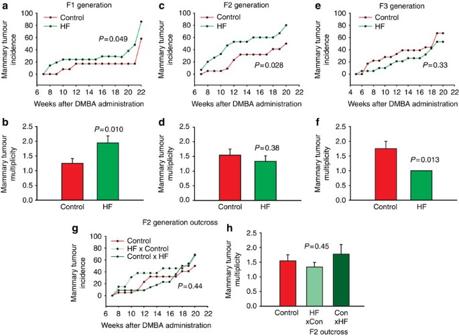Figure 1: Multigenerational effect of maternal HF diet. (a,c,e) Mammary tumour incidence (%) in F1 (control:n=12, HF:n=21), F2 (control:n=22, HF:n=15) and F3 (control:n=18, HF:n=19) generation female offspring of Sprague–Dawley rat mothers (F0) fed a HF diet or a control diet during gestation. (b,d,f) Mammary tumour multiplicity (mean±s.e.m.) in F1 (control:n=7, HF:n=18), F2 (control:n=11, HF:n=12) and F3 (control:n=12, HF:n=10) generation female offspring of Sprague–Dawley rat mothers (F0) fed a HF or a control diet during gestation. (g,h) Mammary tumour incidence (control:n=22, HF×control:n=13, control×HF:n=22) and tumour multiplicity (control:n=11, HF×control:n=9, control×HF:n=15) in F2 generation female (HF×Con) and male (Con×HF) outcrosses. Significant differences versus the control group were determined as follows: log-rank test (tumour incidence),t-test (tumour multiplicty) and one-way ANOVA followed by Dunn'spost-hoctest (outcross groups tumour multiplicity).P<0.05 is considered significant; exactP-values are shown in each plot. Figure 1: Multigenerational effect of maternal HF diet. ( a , c , e ) Mammary tumour incidence (%) in F1 (control: n =12, HF: n =21), F2 (control: n =22, HF: n =15) and F3 (control: n =18, HF: n =19) generation female offspring of Sprague–Dawley rat mothers (F0) fed a HF diet or a control diet during gestation. ( b , d , f ) Mammary tumour multiplicity (mean±s.e.m.) in F1 (control: n =7, HF: n =18), F2 (control: n =11, HF: n =12) and F3 (control: n =12, HF: n =10) generation female offspring of Sprague–Dawley rat mothers (F0) fed a HF or a control diet during gestation. ( g , h ) Mammary tumour incidence (control: n =22, HF×control: n =13, control×HF: n =22) and tumour multiplicity (control: n =11, HF×control: n =9, control×HF: n =15) in F2 generation female (HF×Con) and male (Con×HF) outcrosses. Significant differences versus the control group were determined as follows: log-rank test (tumour incidence), t -test (tumour multiplicty) and one-way ANOVA followed by Dunn's post-hoc test (outcross groups tumour multiplicity). P <0.05 is considered significant; exact P -values are shown in each plot. 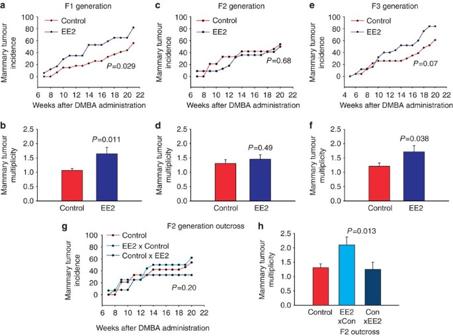Figure 2: Transgenerational effect of maternal EE2-supplemented diet. (a,c,e) Mammary tumour incidence (%) in F1 (control:n=27, EE2:n=17), F2 (control:n=24, EE2:n=22) and F3 (control:n=23, EE2:n=25) generation female offspring of Sprague–Dawley rat mothers (F0) fed a EE2-supplemented diet or a control diet during gestation. (b,d,f) Mammary tumour multiplicity (mean±s.e.m.) in F1 (control:n=15, EE2:n=14), F2 (control:n=13, EE2:n=11) and F3 (control:n=14, EE2:n=21) generation female offspring of Sprague–Dawley rat mothers (F0) fed EE2 or a control diet during gestation. (g,h) Mammary tumour incidence (control:n=24, EE2×control:n=16, control×EE2:n=12) and tumour multiplicity (control:n=13, HF×control:n=10, control×HF:n=4) in F2 generation female outcross (EE2×Con) and male (Con×EE2) outcrosses. Significant differences versus the control group were determined as follows: log-rank test (tumour incidence),t-test (tumour multiplicty) and one-way ANOVA followed by Dunn'spost-hoctest (outcross groups tumour multiplicity).P<0.05 is considered significant; exactP-values are shown in each plot. Full size image Figure 2: Transgenerational effect of maternal EE2-supplemented diet. ( a , c , e ) Mammary tumour incidence (%) in F1 (control: n =27, EE2: n =17), F2 (control: n =24, EE2: n =22) and F3 (control: n =23, EE2: n =25) generation female offspring of Sprague–Dawley rat mothers (F0) fed a EE2-supplemented diet or a control diet during gestation. ( b , d , f ) Mammary tumour multiplicity (mean±s.e.m.) in F1 (control: n =15, EE2: n =14), F2 (control: n =13, EE2: n =11) and F3 (control: n =14, EE2: n =21) generation female offspring of Sprague–Dawley rat mothers (F0) fed EE2 or a control diet during gestation. ( g , h ) Mammary tumour incidence (control: n =24, EE2×control: n =16, control×EE2: n =12) and tumour multiplicity (control: n =13, HF×control: n =10, control×HF: n =4) in F2 generation female outcross (EE2×Con) and male (Con×EE2) outcrosses. Significant differences versus the control group were determined as follows: log-rank test (tumour incidence), t -test (tumour multiplicty) and one-way ANOVA followed by Dunn's post-hoc test (outcross groups tumour multiplicity). P <0.05 is considered significant; exact P -values are shown in each plot. Full size image Effects of HF or EE2 exposure on pregnant F0 dams on mammary cancer risk in the F2 and F3 generations were then examined. In the HF granddaughters (F2 generation), mammary tumour incidence ( P =0.028, log-rank test), but not multiplicity ( P =0.38, t -test), was higher compared with the control group ( Fig. 1c,d ). Mammary tumour incidence did not differ ( P =0.33, log-rank test) between the control and HF great-granddaughters (F3 generation); however, tumour multiplicity was lower ( P =0.013, t -test) in the HF offspring compared with controls ( Fig. 1e,f ). In the EE2 granddaughters (F2 generation), neither tumour incidence ( P =0.68, log-rank test) nor multiplicity ( P =0.49, t -test) was statistically different from the controls ( Fig. 2c,d ). However, EE2 great-granddaughters (F3 generation) had significantly higher tumour multiplicity ( P =0.038, t -test) compared with controls. Mammary tumour incidence was also higher in the EE2 F3 generation, but this difference was not statistically significant ( P =0.07, log-rank test; Fig. 2e,f ) compared with controls. The time to mammary tumour appearance (tumour latency) was not significantly different among the three experimental groups in any of the generations studied ( Supplementary Figs S4 and S5 ). Histopathological analysis indicated that the majority of mammary tumours across all three groups were malignant (adenocarcinomas or solid carcinomas). To investigate whether mammary cancer risk could be transmitted either through the female or male lineages, we mated F1 unexposed males to F1 exposed females or F1 unexposed females to F1 exposed males ( Supplementary Fig. S1b ). Mammary tumour incidence was higher in both HF F2 outcross groups (HF (female)×Con (male): 68%; and Con (female)×HF (male): 69%) compared with controls (50%), but did not reach statistical significance ( P =0.44, log-rank test; Fig. 1g ). Still, these results imply that the effects of HF in utero exposure on mammary cancer risk may be transmitted through both the female or male germ lines. In contrast, EE2 outcross experiments showed a striking difference based on gender of the exposed parent, as only 33% of offspring resulting from Con (female)×EE2 (male) breeding developed mammary tumours, whereas 62% of the EE2 (female)×Con (male) offspring developed mammary tumours ( P =0.20, log-rank test; Fig. 2g ). Tumour multiplicity was also significantly higher in the EE2 (female)×Con (male) outcross offspring compared with controls ( P =0.013, one-way ANOVA; Fig. 2h ). Thus, unlike HF, EE2 exposure had an opposite effect on developing male and female fetuses regarding their ability to transmit susceptibility to mammary cancer to their offspring. Mammary gland morphology in F1–F3 HF and EE2 generations Both HF and EE2 in utero exposures have been shown to alter mammary gland morphology [4] , mainly by increasing the number of terminal end buds (TEBs). These undifferentiated mammary structures are the sites of malignant transformation in rat mammary glands [26] , and corresponding structures in human breasts [26] . We examined whether these effects persisted in the F2 and F3 generation offspring ( Fig. 3a–f ). On PND 21, before puberty, ( Fig. 3c,e ), the number of TEBs was increased in the mammary glands of both HF and EE2 daughters (F1; P =0.032, t -test and P =0.033, t -test, respectively) and granddaughters (F2; P =0.004, t -test and P =0.006, t -test, respectively) compared with control offspring. However, in the great-granddaughters (F3), increase in the number of TEBs was only seen in the offspring of EE2-exposed dams ( P =0.014, t -test). On PND50, at sexual maturity, ( Fig. 3d,f ), the number of TEBs was increased in mammary glands of daughters (F1; P =0.039, t -test) and granddaughters (F2; P =0.044, t -test), but not great-granddaughters (F3), of HF-exposed dams. Although a small increase in TEB number on PND50 was observed in the EE2 offspring, compared with controls, the difference was not significant in any generation. Our results suggest, nonetheless, that an increase in TEB number was closely linked to increased mammary tumourigenesis. 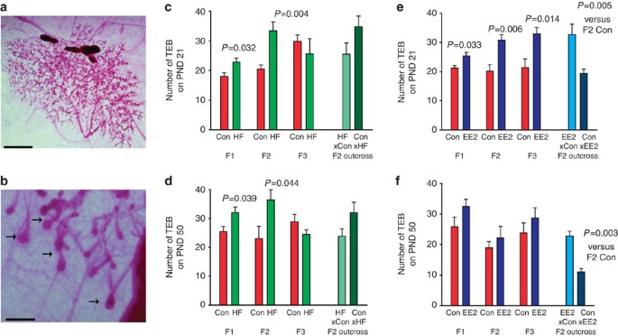Figure 3: Mammary gland morphology in HF or EE2 offspring. (a) Histological depiction of the fourth abdominal rat mammary gland on PND 21 and (b) terminal end buds (TEBs; indicated by arrows). (c) Number of TEBs on PND21 in F1 (control, HF:n=5), F2 (control:n=6, HF:n=5; outcrosses:n=6) and F3 (control, HF:n=5) generation female offspring of Sprague–Dawley rat mothers (F0) fed HF or a control diet during gestation. (d) Number of TEBs on PND50 in F1 (control, HF:n=5), F2 (control:n=6, HF:n=5, outcrosses:n=5) and F3 (control:n=6, HF:n=5) generation female offspring of Sprague–Dawley rat mothers (F0) fed HF or a control diet during gestation. (e) Number of TEBs on PND21 in F1 (control:n=5, EE2:n=6), F2 (control:n=6, EE2:n=5; outcrosses:n=5) and F3 (control, EE2:n=6) generation female offspring of Sprague–Dawley rat mothers (F0) fed EE2 or a control diet during gestation. (f) Number of TEBs on PND50 in F1 (control, EE2:n=6), F2 (control, EE2:n=5; outcrosses:n=6) and F3 (control:n=5, EE2:n=6) generation female offspring of Sprague–Dawley rat mothers (F0) fed EE2 or a control diet during gestation. All values are expressed as the mean±s.e.m. Significant differences versus the control group were determined as follows:t-test (HF, EE2) and one-way ANOVA (outcross groups) followed by Holm-Sidakpost-hoctest.P<0.05 is considered significant; exactP-values are shown in each plot. LN, lymph node; scale bars, 3 mm (a) and 0.5 mm (b). Figure 3: Mammary gland morphology in HF or EE2 offspring. ( a ) Histological depiction of the fourth abdominal rat mammary gland on PND 21 and ( b ) terminal end buds (TEBs; indicated by arrows). ( c ) Number of TEBs on PND21 in F1 (control, HF: n =5), F2 (control: n =6, HF: n =5; outcrosses: n =6) and F3 (control, HF: n =5) generation female offspring of Sprague–Dawley rat mothers (F0) fed HF or a control diet during gestation. ( d ) Number of TEBs on PND50 in F1 (control, HF: n =5), F2 (control: n =6, HF: n =5, outcrosses: n =5) and F3 (control: n =6, HF: n =5) generation female offspring of Sprague–Dawley rat mothers (F0) fed HF or a control diet during gestation. ( e ) Number of TEBs on PND21 in F1 (control: n =5, EE2: n =6), F2 (control: n =6, EE2: n =5; outcrosses: n =5) and F3 (control, EE2: n =6) generation female offspring of Sprague–Dawley rat mothers (F0) fed EE2 or a control diet during gestation. ( f ) Number of TEBs on PND50 in F1 (control, EE2: n =6), F2 (control, EE2: n =5; outcrosses: n =6) and F3 (control: n =5, EE2: n =6) generation female offspring of Sprague–Dawley rat mothers (F0) fed EE2 or a control diet during gestation. All values are expressed as the mean±s.e.m. Significant differences versus the control group were determined as follows: t -test (HF, EE2) and one-way ANOVA (outcross groups) followed by Holm-Sidak post-hoc test. P <0.05 is considered significant; exact P -values are shown in each plot. LN, lymph node; scale bars, 3 mm ( a ) and 0.5 mm ( b ). Full size image We also assessed changes in mammary gland morphology in the outcross offspring ( Fig. 3c–f ). On PND21, mammary glands of Con (female)×HF (male) outcross offspring ( P =0.005, one-way ANOVA), but not HF (female)×Con (male) offspring ( P =0.654, one-way ANOVA), had a higher number of TEBs than the controls. No differences in the number of TEBs were observed between both HF outcross groups and the control group on PND50. Mammary glands of the EE2 (female)×Con (male) outcross offspring also had a significantly higher number of TEBs ( P =0.005, one-way ANOVA) on PND21, but not on PND50 ( P =0.110, one-way ANOVA). Lower number of TEBs was seen on PND50 in the Con (female)×EE2 (male) group, compared with the controls ( P =0.003, one-way ANOVA). Mammary glands from all three generations of offspring were also evaluated for mammary differentiation and ductal elongation ( Supplementary Figs S6 and S7 ). However, no effects of maternal exposure to HF or EE2 on neither of those end points were observed in the offspring's mammary tissue compared with the control group. Mammary DNMT expression in F1–F3 HF and EE2 generations Transgenerational inheritance of disease may be mediated by alterations in DNA methylation [27] , [28] . After DNA replication, DNMT1 methylates the CpG sites on the daughter DNA strand to maintain the parental pattern of methylation [18] , [29] , and is also involved in de novo methylation [17] , [30] , along with DNMT3A and DNMT3B, the two major de novo methyltransferases [18] . We determined whether HF and EE2 exposures during pregnancy affected mRNA expression of Dnmt1 , Dnmt3a and Dnmt3b in the mammary glands of F1–F3 generations on PND50 ( Fig. 4a–f ). Both HF and EE2 in utero exposures increased the levels of Dnmt1 mRNA in F1 generation mammary glands ( P <0.001, two-way ANOVA, for HF and EE2), and this increase persisted to F2 ( P =0.003, two-way ANOVA) and F3 ( P =0.008, two-way ANOVA) generation in the EE2 but not in the HF offspring ( Fig. 4a,d ). Similarly, mammary mRNA levels of Dnmt3a and Dnmt3b were increased in the F2 ( P =0.005, two-way ANOVA) ( Fig. 4e ) and F3 ( P =0.049, two-way ANOVA; Fig. 4f ) generations of the EE2 offspring, respectively, but were not altered in the HF offspring ( Fig. 4b,c ). 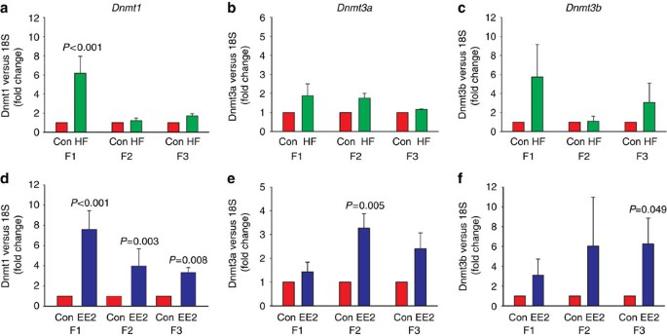Figure 4: Effects of maternal HF or EE2 diet on methyltransferases expression. (a–c)Dnmt1,Dnmt3aandDnmt3bmRNA expression on PND50 in rat mammary glands of F1 (control:n=6, HF:n=5), F2 (control:n=5, HF:n=4) and F3 (control:n=5, HF:n=3) generation female offspring of Sprague–Dawley rat dams (F0) fed HF or control (Con) diet during gestation. (d–f)Dnmt1,Dnmt3aandDnmt3bmRNA expression on PND50 in rat mammary glands of F1 (control, EE2:n=6), F2 (control:n=5, EE2:n=6) and F3 (control, EE2:n=5) generation female offspring of Sprague–Dawley rat dams (F0) fed EE2 or control diet during gestation. Quantitative real-time PCR (qPCR) and absolute quantification method was used.Dnmt1,Dnmt3aandDnmt3bexpression of each sample was normalized to rRNA 18S expression. All data are mean±s.e.m. of two independent experiments performed in triplicates. Significant differences versus the control group were determined by two-way ANOVA (after log-transform) followed by Holm-Sidakpost-hoctest.P<0.05 is considered significant; exactP-values are shown in each plot. Figure 4: Effects of maternal HF or EE2 diet on methyltransferases expression. ( a – c ) Dnmt1 , Dnmt3a and Dnmt3b mRNA expression on PND50 in rat mammary glands of F1 (control: n =6, HF: n =5), F2 (control: n =5, HF: n =4) and F3 (control: n =5, HF: n =3) generation female offspring of Sprague–Dawley rat dams (F0) fed HF or control (Con) diet during gestation. ( d – f ) Dnmt1 , Dnmt3a and Dnmt3b mRNA expression on PND50 in rat mammary glands of F1 (control, EE2: n =6), F2 (control: n =5, EE2: n =6) and F3 (control, EE2: n =5) generation female offspring of Sprague–Dawley rat dams (F0) fed EE2 or control diet during gestation. Quantitative real-time PCR (qPCR) and absolute quantification method was used. Dnmt1 , Dnmt3a and Dnmt3b expression of each sample was normalized to rRNA 18S expression. All data are mean±s.e.m. of two independent experiments performed in triplicates. Significant differences versus the control group were determined by two-way ANOVA (after log-transform) followed by Holm-Sidak post-hoc test. P <0.05 is considered significant; exact P -values are shown in each plot. Full size image DNA methylation patterns in F1–F3 EE2 offspring's mammary gland We then determined whether the increase in Dnmt1 and Dnmt3a/3b expression in the mammary glands of EE2 offspring was associated with differential DNA methylation patterns by using Methyl-CpG Binding domain-based Capture and sequencing (MDBCap-seq) method (data accession code GSE40251). We developed a statistical approach, namely identification of significant inheritable methylation alterations (ISIMA), to examine whether any promoter regions that were differentially methylated between control and EE2 offspring in F1, F2 or F3 generations were common across all three generations. This analysis resulted in the identification of 375 differentially methylated gene promoter regions across the 21 chromosomes, among which 214 were hypermethylated and 161 are hypomethylated ( Fig. 5a and Supplementary Fig. S8 ) in the F1–F3 generation EE2 offspring. Further analysis showed that certain hypermethylated promoter regions ( Fig. 5b ) were associated with polycomb group target genes (PcTGs): Pax6 , Runx3 , Foxe3 , Gata4 and Vgf . PcTGs control stem cell differentiation in normal cells, and are frequently dysregulated in cancer cells [31] , [32] , [33] , [34] . 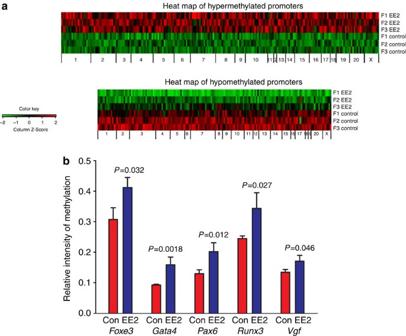Figure 5: Differential promoter methylation in mammary glands of EE2 offspring. (a) Heat maps of differentially methylated gene promoter regions in EE2 offspring (green,n=3) compared with controls (red,n=3). Hypermethylation and hypomethylation are presented separately. MBDCap-seq method was used to access DNA methylation levels. (b) Promoter methylation levels of the polycomb target genes (PcTGs)Foxe3,Gata4,Pax6,Runx3andVgfon PND50 rat mammary glands of F1–F3 generation female offspring of Sprague–Dawley rat dams (F0) fed EE2 or control diet during gestation. Data are presented as relative intensity of methylation (mean±s.e.m.,n=3 per group), ISIMA statistical approach (see Methods section for details).P<0.05 is considered significant; exactP-values are shown in each plot. Figure 5: Differential promoter methylation in mammary glands of EE2 offspring. ( a ) Heat maps of differentially methylated gene promoter regions in EE2 offspring (green, n =3) compared with controls (red, n =3). Hypermethylation and hypomethylation are presented separately. MBDCap-seq method was used to access DNA methylation levels. ( b ) Promoter methylation levels of the polycomb target genes (PcTGs) Foxe3 , Gata4 , Pax6 , Runx3 and Vgf on PND50 rat mammary glands of F1–F3 generation female offspring of Sprague–Dawley rat dams (F0) fed EE2 or control diet during gestation. Data are presented as relative intensity of methylation (mean±s.e.m., n =3 per group), ISIMA statistical approach (see Methods section for details). P <0.05 is considered significant; exact P -values are shown in each plot. Full size image Findings obtained in this study indicate that maternal exposure to HF or EE2 during pregnancy increases mammary cancer risk in multiple generations of offspring. We observed that maternal HF diet increases mammary cancer risk in the daughters and granddaughters. Maternal EE2 exposure increased the risk in three consecutive generations (daughters, granddaughters and great-granddaughters), indicating that the effects are transgenerational for the maternal EE2 exposure, but multigenerational for the maternal HF exposure. Our outcross experiments suggested that increased breast cancer risk in granddaughters can be equally transmitted through in utero HF-exposed fathers or mothers, but this effect was not transgenerational as the F3 generation (great-granddaughters) did not exhibit an increase in mammary cancer risk. A different pattern of inheritance in offspring of dams exposed to EE2 during pregnancy was revealed by outcross experiments: breast cancer risk in granddaughters was determined by whether their mother (increased risk) or father (reduced risk) had been exposed in utero to EE2. These opposing changes may explain why no difference in mammary cancer risk was seen in the F2 generation offspring when both parents had been exposed to EE2 in utero . The breast cancer risk-lowering effect on F1 EE2 male germ line, however, was transient and not transgenerational, because F3 generation females, produced by mating F2 EE2 females with F2 EE2 males, exhibited increased mammary tumour susceptibility. Our findings indicating a difference in mediation of effects of EE2 exposure through female and male germ lines are in agreement with other reports showing that certain in utero exposures have opposite outcomes if transmitted through the male or female germ line. For instance, prenatal under-nutrition leads to reduced birth weights in the second generation offspring of exposed males, but to overweight in the offspring of exposed females [35] . Differences in inheritance through the male and female germ lines in the F2 EE2 generation likely reflect the fact that, in females, germ cells mature before birth, whereas in males these cells are only produced after puberty onset [36] . In both genders, primordial germ cells enter genital ridges on gestation day 10.5. By gestation day 12.5, the cells enter a premeiotic stage in mice [37] and undergo rapid DNA demethylation and sex-specific de novo methylation [38] . In male mice, the primordial cells then undergo mitotic arrest until they start proliferating again at puberty. Premeiotic cells in the female genital ridge, in contrast, enter meiotic prophase as oocytes and reach full maturity as germ cells at the time of birth [39] . Two recent studies show that transmission of DNA methylation occurs mainly through maternal gametes [40] , [41] . Global DNA demethylation, followed by cell- and gender-specific remethylation, occurs twice during fetal development: first in the fertilized egg and then in primordial germ cells when they reach genital ridge. Thus, the multigenerational and transgenerational effects on mammary tumourigenesis of the maternal HF and EE2-supplemented diets, respectively, may be caused by the different durations of these in utero exposures. The HF diet was fed to pregnant dams before conception and throughout pregnancy, whereas the EE2-supplemented diet was fed from day 14 to 20 of pregnancy, as an earlier EE2 exposure would disrupt pregnancy. It is possible that in order for breast cancer risk to be transmitted in a transgenerational manner, the exposures need to occur within a certain window of development, as shown for other diseases [22] . Mammary gland levels of Dnmt1 mRNA were increased in all three EE2 generations, but only in F1 HF generation. Our results are in agreement with other studies showing that in utero exposures to endocrine disruptors alter the expression of DNA methyltransferases in adult target tissues [19] , [20] , [21] . In addition, our results suggest that an increase in mammary cancer risk following maternal exposure to EE2 during pregnancy (F0 dams) may involve an increase in Dnmt1 in each generation of offspring. Further studies will be needed to elucidate how the expression of Dnmt genes in mammary tissue is regulated in the context of in utero oestrogenic exposure, and how these changes are transmitted from one generation to another. The global methylation analysis identified 375 differentially hyper- or hypomethylated gene promoter regions in mammary glands of EE2 daughters, granddaughters and great-granddaughters, hinting at an epigenetic transgenerational effect of EE2. Some of the hypermethylated promoter regions involve the PcTGs Pax6, Runx3, Foxe3, Gata4 and Vgf. These genes regulate stem cell differentiation and are often methylated in these [34] , [42] and in cancer cells [31] , [33] , [43] . The epigenetic trait observed in the EE2 offspring might have been induced and maintained by high levels of Dnmt1, Dnmt3a and Dnmt3b . However, whether the changes in DNA methylation are inherited through gametes or re-established in each generation needs further verification. In addition, it remains to be determined whether the relationship between increased breast cancer risk and differential mammary gland DNA methylation in the EE2 offspring is a causal one or simply an association. It is also possible that other epigenetic mechanisms, such as aberrant histone modification and changes in microRNA expression are involved in mediating the transgenerational effects of EE2 and multigenerational effects of HF on breast cancer risk, but this remains to be investigated. Our results show that an increase in TEB number was closely linked to increased risk of mammary tumourigenesis. These undifferentiated mammary structures are the sites of malignant transformation in the rat mammary gland [26] ; the corresponding structures in the human breast are the terminal ductal lobular units [44] . Studies have shown that higher number of TEBs correlates with higher risk of mammary cancer [26] . Alteration in TEB numbers may also reflect epigenetic modifications in the mammary tissue [45] . In cultures of human mammary cells, for instance, epithelial differentiation is regulated by the expression of genes involved in chromatin remodelling and DNA methylation [46] . This study demonstrates, for the first time, that maternal dietary exposure to HF directly affects two consecutive generations of offspring and causes a multigenerational increase in breast cancer risk, whereas maternal dietary exposure to EE2 during pregnancy initiates a transgenerational increase in the offspring's breast cancer risk that persists up to three consecutive generations and is associated with changes in the DNA methylation machinery and DNA methylation patterns. We did not investigate whether the maternal exposures caused mutations or other genetic alterations in the offspring. However, this is unlikely because no genetic abnormalities have been found in DES daughters [47] and most familial breast cancer cases exhibit no known mutations [1] . If confirmed in humans, our findings represent a novel perspective on how breast cancer risk can be transmitted across generations and could have marked repercussions for breast cancer prevention and treatment. This study also has important public health implications, as intake of HF diets and chronic exposure to low levels of EDCs found in foods and drinking water can lead to adverse effects on human health [48] beyond a single generation. Animals and breeding Sprague–Dawley rats were used in all experiments. Animals were housed in a temperature- and humidity-controlled room under a 12-h light–dark cycle. All animal procedures were approved by the Georgetown University Animal Care and Use Committee, and the experiments were performed following the National Institutes of Health guidelines for the proper and humane use of animals in biomedical research. The F1, F2 and F3 generations were obtained as described below. Only the original pregnant dams (F0) carrying the F1 generation received experimental dietary exposures. To generate the F1 rats, two females and 1 male per cage were mated. For in utero HF exposure, pregnant rat dams (F0) were divided into two groups: AIN93G control diet (17% energy from fat) and HF diet (HF, 43% energy from fat). Both groups were fed the experimental diets for the extension of the pregnancy. The main source of fat in the HF diet was corn oil (n-6 PUFA). For in utero EE2 exposure, pregnant rat dams (F0) were divided into two groups: AIN93G control diet (17% energy from fat) and EE2-supplemented diet (EE2, 0.1 p.p.m.). The composition of the EE2-supplemented diet was similar to the control diet, except for the addition of 0.1 p.p.m. of EE2. The control group was on the control diet for the extent of the pregnancy, whereas the EE2 group was fed the control diet from days 1 to 13 and the EE2-supplemented diet from days 14 to 20 of gestation. One day before they delivered, all rat dams were switched to the control AIN93G diet. Pregnant dams were weighed once a week to monitor changes in weight gain. Birth weight of pups and number of pups per litter were recorded. To avoid litter-effect, pups were cross-fostered 1–2 days after dams gave birth. Pups from two to four dams were pooled and housed in a litter of eight to ten pups per nursing dam (which had the same dietary/hormonal exposure during pregnancy as the pups' mothers). All pups were weaned on PND 21. The F1 female offspring was used to breed subsequent generations, study mammary tumourigenesis and mammary gland morphology. To obtain the F2 generation, F1-exposed (EE2 or HF diet) female rats were mated with F1-exposed males. The control groups (AIN93G control diet) were mated in the same manner. Pregnant dams were fed a standard AIN93G diet throughout pregnancy. No sibling mating was carried out. Monitoring of pregnancy, pups cross-fostering and weaning was carried out as described for the F1 generation. Outcross experiments were also performed to determine whether the transgenerational effect on mammary cancer risk is transmitted to the female or male germ line or both. F1 females exposed to EE2 (EE2 female) or HF (HF female) diet in utero were crossed with untreated control males (Con males). The reverse outcross was also performed: F1 males exposed to EE2 (EE2 male) or HF (HF male) diet in utero were crossed with untreated control females (Con female). To obtain the F3 generation, F2 females and F2 males from each exposure group were mated in the same manner as described above to produce the F3 generation. Pregnant dams were fed a standard AIN93G diet throughout pregnancy. Mammary gland harvesting On PND 21 and 50, mammary glands of F1, F2 and F3 generation female pups were collected and used to study mammary gland morphology as described below. Mammary gland morphology The fourth abdominal mammary glands obtained from 21- and 50-day-old F1–F3 offspring were dissected, stretched onto a slide, placed in a fixative solution and stained with a carmine aluminium solution to prepare whole mounts [49] . Whole mounts were examined under the microscope and evaluated to assess the number of TEBs. In addition, whole mounts were evaluated for ductal elongation and differentiation. On PND 21, ductal elongation was measured, using a ruler, as the distance (in centimeters) from the nipple to the end of epithelial tree. Mammary gland differentiation was assessed by scoring the number of alveolar buds (ABs) type 1 and type 2. The score values (0–5) from AB1 and AB2 were added for a final differentiation score (0–10). On PND 50, ductal elongation was measured as the distance (in centimeters) from the tip of the epithelial tree to the end of fat pad. Mammary gland differentiation was assessed by scoring the number of ABs type 1 and 2 and lobules. The average score values (0–5) from AB1 and AB2 were added to the lobule score values (0–5) for a final differentiation score (0–10). Results were analysed by t -test (or appropriate non-parametric test) and one-way analysis of variance (ANOVA; when comparing outcross groups in F2 generation). Where appropriate, between groups comparisons were done by Holm-Sidak post-hoc test. Mammary tumourigenesis Mammary tumours were induced in 50-day-old (±2 days) F1, F2 and F3 generation females by administration of oral gavage of 10 mg of 7,12-dimethylbenz[a]anthracene (DMBA; Sigma, St Louis, MO) in 1 ml of peanut oil [50] . Tumourigenesis (incidence and multiplicity) was monitored for 20 weeks. Rats were examined for mammary tumours by palpation once per week, starting on week 3 post-DMBA and continued for 20 weeks post DMBA. Tumour growth was measured using a caliper and the length, width, and height of each tumour were recorded. The end points for data analysis were (i) latency to tumour appearance, (ii) the number of animals with tumours (tumour incidence) and (iii) the number of tumours per animal (tumour multiplicity). During the follow-up, those animals in which tumour burden approximated 10% of total body weight were killed, as required by our institution. Differences in tumour latency and multiplicity were tested by t -test (or appropriate non-parametric test) and one-way ANOVA (where appropriate between groups comparisons were done by Dunn's post-hoc test). Kaplan–Meier survival curves were used to compare differences in tumour incidence, followed by the log-rank test. Tumour histopathology was analysed by a veterinary pathologist, from ARUP laboratories, Salt Lake City, Utah. Complementary DNA synthesis and quantitative real-time PCR analysis Two hundred nanograms of total RNA per sample was used as a template for random primed cDNA synthesis with a recombinant Moloney murine leukaemia virus reverse transcriptase (TaqMan MultiScribe Reverse Transcriptase and RT–PCR Reagents, Applied Biosystems, Roche, New Jersey, USA), according to manufacturer's instructions. An RT enzyme-minus control reaction was also included. The cDNA samples were then used as templates for quantitative real-time PCR analysis with specific primers ( Supplementary Table S1 ) for the target gene [51] , [52] , rat Dnmt1, Dnmt3a and Dnmt3b using QuantiTect SYBR green PCR kit (Qiagen, Valencia, CA) and an ABI Prism 7900 Sequence Detection System. Each sample was run in triplicate, and the quantitative PCR (qPCR) run was repeated twice. Absolute gene expression levels were determined using SDS2.3 software (Applied Biosystems) and the standard curve method. Concentration of each sample was normalized to the reference gene 18S rRNA [53] , and averages of the three runs are shown. Differences in Dnmt1 , Dnmt3a and Dnmt3b mRNA expression levels were tested by two-way ANOVA (after log-transformation), followed by Holm-Sidak post-hoc test. Genome-wide methylation analysis Genomic DNA was isolated using the Wizard Genomic DNA Purification Kit (Promega, Madison, WI) following the manufacturer's instructions. Methylated DNA was eluted by the MethylMiner Methylated DNA Enrichment Kit (Invitrogen) according to the manufacturer's protocol. Briefly, 1 μg of genomic DNA was sheared by sonication and captured by MBD proteins. Methylated DNA was eluted, precipitated and resuspended in TE buffer. Using the eluted DNA, MBDCap libraries were generated [54] . MBDCap coupled with massively parallel sequencing (MBDCap seq) libraries were sequenced using the Illumina Genome Analyzer II (GA II) as per manufacturer's instructions. Image analysis and base calling were performed with the standard Illumina pipeline. Sequencing reads were mapped by ELAND algorithm. Identification of methylation alterations Statistical analyses of methylation patterns across generations were focused on the gene promoter regions defined as up to 5,000 base pairs upstream of transcription starting site. The CpG islands within the promoter regions were identified as previously described [55] . To explicitly account for the background rate of random methylations and to distinguish meaningful events from random background methylation, we developed a statistical approach, called ISIMA, for identifying regions of methylation changes more likely to drive cancer risk across generations than would be expected by chance [56] . ISIMA identified significant inheritable methylation changes between EE2 generations through two key steps. First, the method calculated a statistic that involves both the frequency and amplitude of the methylation change with methylation intensity being the counts of mapped methylation short reads within each of the gene promoter regions. Second, it assessed the statistical significance of each promoter methylation change using a positional permutation test that is based on the overall pattern of methylation changes seen across the gene promoter regions. ISIMA revealed a highly concordant inheritability picture involving 375 significant events ( P <0.002), including hypermatylation and hypomethylation changes in gene promoter regions. We also found many significant events ( P <0.05) that are associated with cancer risk genes (PcTGs) on the CpG islands within these promoter regions. Additional description of the statistical analyses can be found in the Supplementary Methods section. Accession codes: The genome-wide methylation data have been deposited in the Gene Expression Omnibus database under accession code GSE40251 . How to cite this article: de Assis, S. et al . High-fat or ethinyl-oestradiol intake during pregnancy increases mammary cancer risk in several generations of offspring. Nat. Commun. 3:1053 doi: 10.1038/ncomms2058 (2012).